Dearomative 1,4-difunctionalization of naphthalenes via palladium-catalyzed tandem Heck/Suzuki coupling reaction Dearomative functionalization reactions represent an important strategy for the synthesis of valuable three-dimensional molecules from simple planar aromatics. Naphthalene is a challenging arene towards transition-metal-catalyzed dearomative difunctionalization reactions. Reported herein is an application of naphthalene as a masked conjugated diene in a palladium-catalyzed dearomative 1,4-diarylation or 1,4-vinylarylation reaction via tandem Heck/Suzuki sequence. Three types of 1,4-dihydronaphthalene-based spirocyclic compounds are achieved in excellent regio- and diastereoselectivities. Key to this transformation is the inhibition of a few competitive side reactions, including intramolecular naphthalenyl C-H arylation, intermolecular Suzuki cross-coupling, dearomative 1,2-difunctionalization, and dearomative reductive-Heck reaction. Density functional theory (DFT) calculations imply that the facile exergonic dearomative insertion of a naphthalene double bond disrupts the sequence of direct Suzuki coupling, leading to the tandem Heck/Suzuki coupling reaction. The observed regioselectivity towards 1,4-difunctionalization is due to the steric repulsions between the introduced aryl group and the spiro-scaffold in 1,2-difunctionalization. Owing to the facile assembly of complex molecules starting from readily available olefins, transition-metal-catalyzed olefin difunctionalization has received considerable attention in past decades [1] , [2] , [3] , [4] , [5] , [6] , [7] , [8] , [9] . In this context, domino transformations involving initial carbometalation of simple alkenes or conjugated dienes and subsequent capture of the in situ generated σ-alkylmetal or π-allyl-metal species has been intensely developed for this purpose (Fig. 1a ) [10] , [11] , [12] , [13] , [14] , [15] , [16] . On the other hand, as disclosed recently by the groups of Lautens [17] , [18] , [19] , [20] , Liang [21] , Yin [22] , [23] , Zhou [24] , Wu [25] , and us [26] , [27] , [28] , [29] , [30] , the application of endocyclic C=C bonds of heteroarenes as non-classic olefins has enabled a number of efficient dearomative difunctionalization reactions of indoles and furans with Pd- or Ni-catalyst [31] . This dearomatizing strategy undoubtedly expands the scope of olefin difunctionalization reaction to arenes and constitutes an important method for the synthesis of valuable three-dimensional molecules from simple planar aromatics [32] , [33] , [34] , [35] , [36] , [37] , [38] . However, the present study is still in its infancy and is limited to reactive heteroarenes, which tend to dearomatization due to their generally lower resonance stabilization energy. It is highly desirable to extend this reaction to additional aromatic compounds, in particular, for those less reactive arenes. Fig. 1: Transition-metal-catalyzed difunctionalization of olefin and arene. a TM-catalyzed difunctionalization of alkene (well-developed) [2] , [9] , [10] , [11] , [12] , [13] , [14] , [15] , [16] . b Dearomative difunctionalization of naphthalene or benzene (unknown). c Dearomative 1,4-diarylation/vinylarylation of naphthalenes via Heck/Suzuki coupling (This work). [M] metal catalyst, Nu nucleophile, L ligand, L′ linker, Ar arene. Full size image Naphthalene and benzene are abundant aromatic molecules while remain much less reactive toward the above-mentioned dearomative difunctionalization reactions [34] , [35] , [36] , [37] , [38] , [39] . When viewing naphthalene as a masked conjugated diene, not only dearomatizing carbometalation but also regioselective and diastereoselective capture of the in situ formed π-allyl-metal species remain challenging (Fig. 1b ). In addition, competitive side reactions including naphthalenyl C–H functionalization and the direct cross-coupling with capturing agents impeded this study. To our knowledge, there has no example reported for the dearomative difunctionalization of naphthalenes through palladium-catalyzed Heck/anionic-capture sequence [40] , [41] , [42] , [43] , [44] , [45] , [46] , [47] , [48] , [49] , [50] . As our interest of dearomatization reactions [26] , [27] , [28] , [29] , [30] , [51] , [52] , [53] , [54] , we report herein a dearomative 1,4-difunctionalization of naphthalenes via intramolecular dearomative Heck arylation or vinylation followed by intermolecular cross-coupling with the π-allyl-palladium species (Fig. 1c ). A range of 1,4-dihydronaphthalene-based spirocycles bearing oxindole, dihydrobenzofuran, or indene subunits are achieved in moderate to excellent yields, which are frequently occurring structural frameworks in natural products and bioactive molecules. Both regioselectivity and remote diastereoselectivity of two newly formed carbocenters at C1 and C4 are well controlled. Key to this reaction relies on the inhibition of a few competitive side reactions, including intramolecular naphthalenyl C–H arylation, intermolecular Suzuki cross-coupling, 1,2-difunctionalization, and dearomative reductive-Heck reaction. DFT calculations reveal the mechanistic basis for the tandem Heck/Suzuki coupling reaction and the controlling factors of chemo- and regioselectivities. 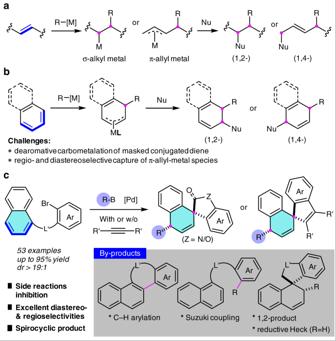Fig. 1: Transition-metal-catalyzed difunctionalization of olefin and arene. aTM-catalyzed difunctionalization of alkene (well-developed)2,9,10,11,12,13,14,15,16.bDearomative difunctionalization of naphthalene or benzene (unknown).cDearomative 1,4-diarylation/vinylarylation of naphthalenes via Heck/Suzuki coupling (This work). [M] metal catalyst, Nu nucleophile,Lligand, L′ linker, Ar arene. Optimization study Our study began with the reaction optimization of N -(2-bromophenyl)- N -methyl-1-naphthamide 1a with phenylboronic acid 2a (Table 1 ). It has turned out that 1,4-product 3a was difficult to be achieved as a series of by-products 4 – 7 were observed in the reaction. As shown in Fig. 2 , initial test in the presence of 5 mol% Pd(dba) 2 , 10 mol% PPh 3 , and 2.5 equiv K 2 CO 3 in toluene led to by-product 4 in 90% NMR (Nuclear Magnetic Resonance) yield via an intermolecular Suzuki cross-coupling (see also entry 1). Not surprisingly, the intramolecular naphthalenyl C–H arylation reaction proceeded smoothly to afford compound 7 in 70% yield in the absence of phenylboronic acid 2a . Although the desired product 3a and by-product 5 were detected in very poor yields, it indicated the occurrence of naphthalene dearomatization. Table 1 Reaction optimization a . Full size table Fig. 2: Initial test with Ph 3 P as ligand. The yields refer to NMR yield using MeNO 2 as an internal standard. dba (1 E ,4 E )-1,5-diphenylpenta-1,4-dien-3-one. Full size image Further ligand evaluation showed that the racemic BINOL ([1,1′-binaphthalene]-2,2′-diol)-derived phosphoramidite L1 provided 3a in a promising yield (16%) along with by-product 5 (7%) derived from dearomative reductive-Heck reaction. Cy 3 P and (EtO) 3 P gave similar results as PPh 3 (entries 2–4). Nevertheless, excellent diastereoselectivity (>19:1) was observed for 3a , whose structure and the relative configuration were determined by X-ray analysis. Encouraged by this result, other racemic phosphoramidites L2 – L4 bearing different substituents on nitrogen atom were examined subsequently (entries 5–7). It was found that steric hindrance of the amino moiety facilitated the formation of 3a . For example, L4 bearing a dicyclohexylamino group led to 3a in 46% yield along with the detection of by-products 4 – 6 (entry 7). Comparable yield of 3a was achieved for L5 containing a spiro-backbone [55] , while compound 4 was the only by-product in this case (entry 8). To further improve the product yield, influence of the base and solvent were then investigated in the presence of ligand L5 (entries 9–13 and 15–18). Gratifyingly, NMR yield of 3a was substantially improved to 83% by employing KF as a base (entry 12), whereas no product or lower yields were observed for Na 2 CO 3 , Cs 2 CO 3 , K 3 PO 4 , and CsF (entries 9–11 and 13). As a comparison, the reaction using L4 as a ligand in the presence of KF base led to 3a in 71% yield (entry 14). Toluene was proved to be the best choice of solvent, although comparable yields were observed in THF, DME, and DMF (entries 15, 16, and 18). Noticeably, the reaction in MeCN led to relatively higher yields for by-products 5 and 7 (entry 17). Elevating the reaction temperature to 140 °C resulted in a slightly improved NMR yield of 3a (86%), which was isolated in 79% yield (entry 20). Switching PhB(OH) 2 to Ph 4 BNa further improved the isolated yield to 83%, along with trace amount of by-product 4 and 1,2-isomer 6 (entry 21). It is noting that lower enantioselectivities of the product were observed when the corresponding chiral ligands were used (entry 4 ( S )- L1 , 16% ee; entry 5 ( R )- L2 , 8% ee; entry 6 ( S )- L3 , 12% ee; entry 7 ( S )- L4 , 11% ee; entry 20 ( R )- L5 , 5% ee). As shown in entries 22 and 23, the influence of halides in the substrate 1 was investigated. Product 3a was obtained in 89% NMR yield for iodo-substrate and 27% for the chloro-substrate. Substrate scope evaluation With the optimal conditions in hand, the scope of amide 1 was then evaluated (Fig. 3 ). Good yields and excellent diastereoselectivity (>19:1) were detected for the substrates bearing an aniline ring with different steric and electronic profiles. A variety of substituents, including Me, MeO, CF 3 , F, Cl, CF 3 O, acetyl, ester, and amide were well tolerated in the reaction. No steric effect was observed in the reactions of substrates bearing substituents ortho to bromide atom and the corresponding products 3b – 3e were achieved in good to excellent yields. In addition to N -methyl substrates, the reaction of N -benzyl substrate delivered product 3u in a higher yield (95%). The reaction was also compatible with a pyridine-derived substrate, which afforded product 3v in 72% yield. Moreover, for the reaction of substrate bearing an extra bromide atom on the naphthalene ring, an unsurprisingly diphenylated product 3x was isolated in 71% yield with excess amount of Ph 4 BNa and KF. Excellent yield was also observed for product 3w containing a methoxy group on naphthalene ring. Interestingly, although Cl atom at C5 of product 3j survived in the reaction, Cl para to bromide coupled with Ph 4 BNa to afford diphenylated product 3y in 58% yield. In these two cases three C–C σ-bonds were generated in one step. Extension of the reaction to 1,4-difunctionalization of benzene was unsuccessful, while excellent yield of 88% was achieved for an antracene-substrate 1z . When a para -MeO-substrate 8 was used, the 1,4-diarylation product 9 was isolated in 51% yield as a major product along with 1,2-product 10 in 22% yield. Fig. 3: Substrate scope of amides. The standard reaction conditions were used, as shown in Table 1 , entry 21. Isolated yield are presented. Full size image Considering the commercial availability of aromatic boronic acids, we then applied them as coupling partners for this 1,4-difunctionalization reaction. 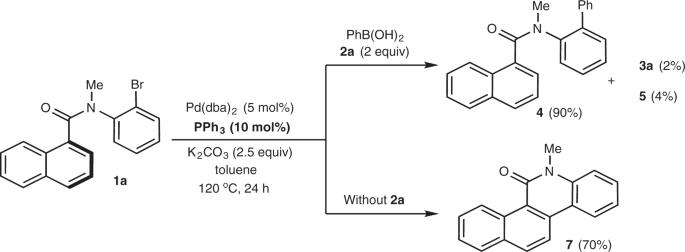Fig. 2: Initial test with Ph3P as ligand. The yields refer to NMR yield using MeNO2as an internal standard. dba (1E,4E)-1,5-diphenylpenta-1,4-dien-3-one. As shown in Table 2 , reactions of 1a with various of boronic acids 2 bearing different substituents, such as Me, F, Cl, CF 3 , and Ph, at o -/ m -/ p -positions of benzene ring proceeded well to afford the desired products in 50-90% yields with excellent diastereoselectivity (>19:1). Noteworthy is that a vinyl moiety bearing on the benzene ring of 2 has no disturbance to the reaction, affording product 3ai in 46% yield (entry 9). Other than 1-naphthamide substrate, the reaction is also compatible with arylether tethered naphthalene 11 . Under the standard conditions, the anticipated 1,4-diarylation product 12 was afforded in 55% yield and with >19:1 diastereomeric ratio (Fig. 4 ). This not only extends the scope of naphthalene, but also provides a reliable synthetic approach to dihydrobenzofuran-derived spirocycle. Table 2 Scope of boronic acids a . Full size table Fig. 4: 1,4-Diarylation of arylether tethered naphthalene 11 . Reaction conditions: 11 (0.2 mmol), Pd(dba) 2 (0.01 mmol), L5 (0.02 mmol), Ph 4 BNa (0.2 mmol), KF (0.5 mmol), toluene (2 mL), 140 °C, 16 h, isolated yield. Full size image Theoretical calculation study To shed light on the reaction mechanism and origins of chemo- and regioselectivities, density functional theory (DFT) calculations were performed using the N -(2-bromophenyl)- N -methyl-1-naphthamide 1a and phenylboronic acid 2a as the model. The computed free energy changes of the tandem Heck/Suzuki reaction (black pathway) and the intermolecular Suzuki cross-coupling reaction (blue pathway) are shown in Fig. 5 . From the Pd L 2 complex, ligand exchange with 1a leads to the arene-coordinated intermediate int1 . Subsequent oxidative addition via TS2 generates the Pd(II) intermediate int3 , which undergoes insertion through TS4 to form the allyl-palladium intermediate int5 . Transmetalation of int5 with PhB(OH) 2 F anion (see Supplementary Fig. 185 for the formation of PhB(OH) 2 F anion) via TS7 irreversibly affords the (allyl)palladium(phenyl) intermediate int8 . Subsequent reductive elimination through TS9 eventually produces the Heck/Suzuki product 3a and regenerates the Pd(0) active catalyst. Alternatively, int3 can also directly undergoes transmetalation with PhB(OH) 2 F anion to form the biarylpalladium(II) intermediate int12 . Subsequent aryl–aryl reductive elimination through TS13 would produce the classic intermolecular Suzuki cross-coupling product 4 . The overall barrier for the formation of Heck/Suzuki product 3a is 1.5 kcal/mol lower than that for the formation of 4 ( TS7 vs TS11 ), indicating that the formation of 3a is more favorable than that of 4 . This is consistent with the experimental results that the ratio of 3a and 4 is 86:8 (Table 1 , entry 20). Therefore, the chemoselectivity-determining transmetalation step differentiates the tandem Heck/Suzuki coupling reaction and the competing classic intermolecular Suzuki cross-coupling. The facile exergonic insertion of pendant naphthalene double bond via TS4 interrupts the sequence of Suzuki cross-coupling and drives the reaction toward the tandem Heck/Suzuki coupling reaction. We have also considered a number of alternative mechanistic pathways, and the details of these unfavorable pathways are included in the Supporting Information (Supplementary Figs. 187 and 188 ). Fig. 5: Theoretical calculations. DFT-computed free energy profiles of the most favorable pathway for the formation of 3a and by-product 4 ( L = L5 ). Full size image Based on the mechanistic model, we next explored the regioselectivity of 1,4- and 1,2-diarylation. The energies and optimized structures of the competing reductive elimination transition states are shown in Fig. 6 (see Supplementary Fig. 188 for the entire DFT-computed Gibbs free energy profile of the regioisomeric 1,2-difunctionalization). TS9 is 3.0 kcal/mol more favorable than TS14 , which is consistent with the experimental observations of 1,4-diarylation as the major product. The 1,2-diarylation is less favorable due to the steric repulsions between the phenyl moiety of the forming C−C bond and the spiro-scaffold. Indeed, replacing the spiro-scaffold with methylene led to a reversed chemoselectivity (see Supplementary Fig. 189 ). This suggested that the intrinsic chemoselectivity favors the 1,2-difunctionalization because of the conjugation in the styrene product, while the steric repulsions overrule the intrinsic preference and favors the 1,4-difunctionalization. Fig. 6: Theoretical calculations. DFT-computed free energies of the regioselectivity-determining reductive elimination transition states ( L = L5 ). Full size image Three-component dearomative reaction We further envisioned a three-component tandem reaction between 1-(2-bromophenyl)naphthalene 13 , alkyne 14 , and sodium tetraarylborates to synthesize indene-derived spirocarbocycles. In this dearomative 1,4-vinylarylation reaction, three C–C bonds would generate in one step through the first insertion of Ar–Pd species to alkyne, the second insertion of the resulting alkenyl–Pd intermediate to naphthalene, and the final transmetalation with tetraphenylborate followed by reductive elimination. 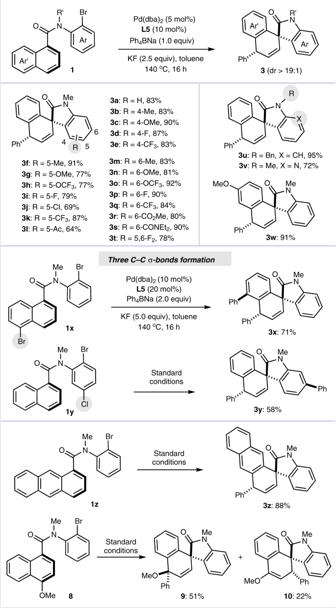Fig. 3: Substrate scope of amides. The standard reaction conditions were used, as shown in Table1, entry 21. Isolated yield are presented. To our delight, under the above optimal conditions, both aryl and alkyl substituted internal alkynes reacted smoothly with naphthalene 13 and Ph 4 BNa, offering the spirocarbocycles 15a – 15i in moderate to good yields with excellent diastereoselectivities (Table 3 , entries 1–9). Effect of the substituents attached on the benzene ring of arylbromides was also tested, which afforded the desired products 15j – 15n in the yields ranging from 55% to 83% (entries 10–13). Table 3 Three-component dearomative 1,4-vinylarylation reaction a . Full size table Scale-up reaction and product transformation To demonstrate the practicality of this protocol, a scale-up reaction was carried out and product 3a was isolated in 87% yield (Fig. 7a ). As shown in Fig. 7b , non-conjugated carbon–carbon double bond of 3a was prone to isomerization in the presence of t BuOK, affording spirooxindole 16 bearing a styrene moiety in 91% yield. Moreover, a Pd/C-catalyzed hydrogenation of alkene with H 2 balloon led to saturated spirocarbocycle 17 in 92% yield. It is noted that compounds 3a , 16 , and 17 are analogs of a patented bioactive molecule for treating pain [56] , which indicates further potential application of the present method. Fig. 7: Scale-up reaction and synthetic transformations. a 1.0 mmol scale-synthesis of product 3a . b Transformations of product 3a . (i) isomerization of carbon–carbon double bond of 3a with t BuOK. (ii) reduction of carbon–carbon double bond of 3a with Pd/C catalyst under H 2 atmosphere. Full size image In summary, an efficient dearomative 1,4-diarylation of naphthalenes has been developed through palladium-catalyzed tandem Heck/Suzuki coupling reaction. A few competitive side reactions are overcome with excellent control of chemo-, regio-, and diastereoselectivities in this reaction. This protocol is further extended to three-component dearomative 1,4-vinylarylation of naphthalenes with alkynes and tetraarylborates. The dearomative 1,4-difunctionalization reaction has provided facile accesses to unique spirocyclic compounds. DFT calculations revealed the reaction mechanism and elucidated the origins of chemo- and regioselectivities. 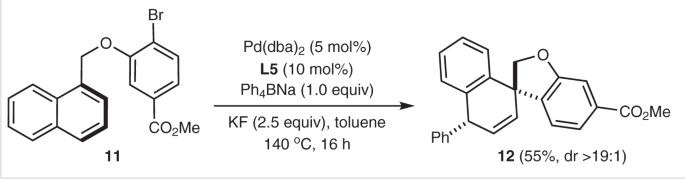Fig. 4: 1,4-Diarylation of arylether tethered naphthalene11. Reaction conditions:11(0.2 mmol), Pd(dba)2(0.01 mmol),L5(0.02 mmol), Ph4BNa (0.2 mmol), KF (0.5 mmol), toluene (2 mL), 140 °C, 16 h, isolated yield. 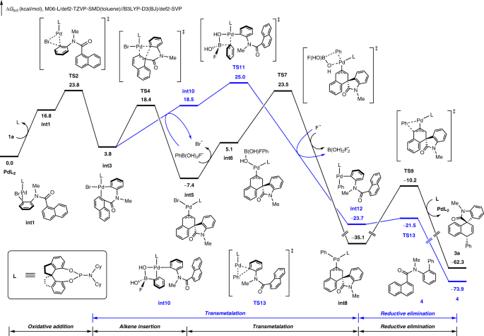Fig. 5: Theoretical calculations. DFT-computed free energy profiles of the most favorable pathway for the formation of3aand by-product4(L=L5). It is the facile exergonic insertion of naphthalene double bond that disrupts the sequence of direct Suzuki coupling, leading to the tandem Heck/Suzuki coupling reaction. The steric repulsions between the aryl group of the forming C−C bond and the spiro-scaffold disfavors the intrinsic regioselectivity toward 1,2-difunctionalization, allowing the observed 1,4-difunctionalization. General procedure for the reaction of 1 , 8 , or 11 To a dried Schlenk tube were added 1 , 8 , or 11 (0.20 mmol), Pd(dba) 2 (5.8 mg, 0.010 mmol), ligand L5 (9.2 mg, 0.020 mmol), NaBPh 4 (68.4 mg, 0.20 mmol) or ArB(OH) 2 (0.40 mmol), KF (29.1 mg, 0.50 mmol) under N 2 . 2.0 mL toluene was then introduced via syringe and the tube was sealed using Teflon cap. 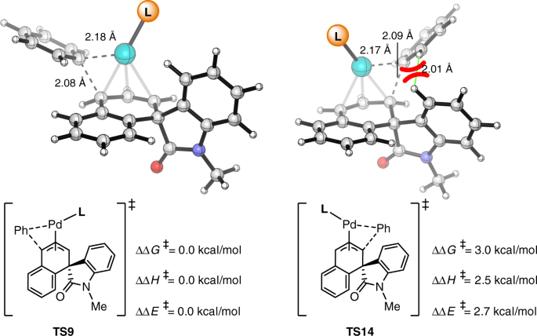Fig. 6: Theoretical calculations. DFT-computed free energies of the regioselectivity-determining reductive elimination transition states (L=L5). 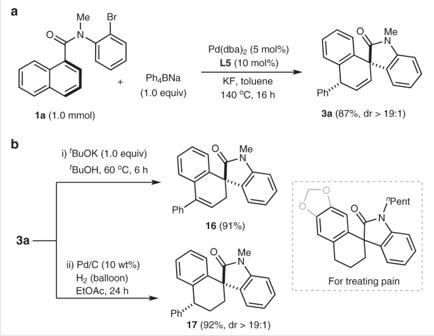Fig. 7: Scale-up reaction and synthetic transformations. a1.0 mmol scale-synthesis of product3a.bTransformations of product3a. (i) isomerization of carbon–carbon double bond of3awithtBuOK. (ii) reduction of carbon–carbon double bond of3awith Pd/C catalyst under H2atmosphere. The mixture was stirred at 140 °C until the starting material was consumed. The solvent was then removed under vacuum and the residue was purified by chromatography on silica gel, eluting with ethyl acetate/petroleum ether to afford the products 3 , 9 , or 12 . General procedure for the reaction of 13 To a dried Schlenk tube were added 13 (0.20 mmol) and 14 (0.30 mmol), Pd(dba) 2 (5.8 mg, 0.010 mmol), ligand L5 (9.2 mg, 0.02 mmol), Ar 4 BNa (0.20 mmol), KF (29.1 mg, 0.50 mmol) under N 2 . 2.0 mL toluene was then introduced via syringe and the tube was sealed using Teflon cap. The mixture was stirred at 140 °C for 16 h. The solvent was then removed under vacuum and the residue was purified by chromatography on silica gel, eluting with dichloromethane/petroleum ether to afford the products 15 .